Inhibition of osteoclastogenesis and inflammatory bone resorption by targeting BET proteins and epigenetic regulation Emerging evidence suggests that RANKL-induced changes in chromatin state are important for osteoclastogenesis, but these epigenetic mechanisms are not well understood and have not been therapeutically targeted. In this study, we find that the small molecule I-BET151 that targets bromo and extra-terminal (BET) proteins that ‘read’ chromatin states by binding to acetylated histones strongly suppresses osteoclastogenesis. I-BET151 suppresses pathologic bone loss in TNF-induced inflammatory osteolysis, inflammatory arthritis and post-ovariectomy models. Transcriptome analysis identifies a MYC-NFAT axis important for osteoclastogenesis. Mechanistically, I-BET151 inhibits expression of the master osteoclast regulator NFATC1 by suppressing expression and recruitment of its newly identified upstream regulator MYC. MYC is elevated in rheumatoid arthritis macrophages and its induction by RANKL is important for osteoclastogenesis and TNF-induced bone resorption. These findings highlight the importance of an I-BET151-inhibited MYC-NFAT axis in osteoclastogenesis, and suggest targeting epigenetic chromatin regulators holds promise for treatment of inflammatory and oestrogen deficiency-mediated pathologic bone resorption. Osteoclasts are bone-resorbing cells important for bone homeostasis and pathological bone resorption [1] , [2] , [3] , [4] , [5] . M-CSF and RANKL are key factors required for differentiation of myeloid lineage cells into osteoclasts. M-CSF promotes proliferation and survival of myeloid cells and induces expression of RANK, the receptor for the key inducer of osteoclastogenesis RANK ligand (RANKL). RANKL drives osteoclast differentiation by activating the NF-κB, MAPK and calcium signalling pathways to induce and activate a transcription factor NFATc1, a master regulator of osteoclastogenesis. RANKL-mediated signalling pathways are well characterized [1] , and RANKL–RANK interactions and downstream signalling pathways have been targeted to treat osteoporosis and other bone diseases. Recently, it has become apparent that RANKL-induced changes in chromatin state of osteoclast precursors are important for osteoclastogenesis [6] , [7] . However, epigenetic mechanisms that regulate osteoclast differentiation have not been well clarified or therapeutically targeted. Epigenetic regulation, which includes modifications of DNA and chromatin, and expression of noncoding RNA, plays an important role in physiological responses and pathological conditions [8] , [9] , [10] . Recent development of drugs that target epigenetic mechanisms, including chromatin states, holds great promise in treating diseases such as cancers [11] , [12] . Bromodomain and extra-terminal (BET) proteins ‘read’ chromatin states by binding to acetylated histones (H-Ac) via bromodomains and recruit additional chromatin regulators to control gene transcription [13] . Small-molecule inhibitors that target the BET family have been generated and inhibition of interaction of BET proteins with H-Ac using small-molecule inhibitors effectively suppresses tumour growth and inflammatory responses in mouse models [13] , [14] , [15] , [16] , [17] , [18] , [19] . These inhibitors show high specificity for their targets, specifically binding the BET family proteins, and minimal systemic toxicity, suggesting a high potential as effective and safe therapeutics [11] , [14] , [15] , [20] . Here, we report that the small-molecule inhibitor I-BET151 that targets BET proteins effectively suppresses RANKL-induced osteoclastogenesis. I-BET151 treatment suppressed in vivo bone loss in post ovariectomy osteoporosis, inflammatory arthritis and TNF-induced osteolysis mouse models. Transcriptome analysis revealed that I-BET151 inhibits NFATc1 expression by suppressing MYC, and we identified a MYC-NFAT axis important for osteoclastogenesis that is targeted by I-BET151. These findings implicate MYC and BET proteins in osteoclastogenesis, and suggest targeting epigenetic chromatin regulators as a new therapeutic approach for controlling inflammatory bone resorption. I-BET151 suppresses osteoclastogenesis in vitro and in vivo We tested the effects of BET bromodomain protein inhibition on osteoclast differentiation. I-BET151 suppressed the differentiation of human and mouse osteoclast precursors (OCPs) into multinucleated tartrate-resistant acid phosphatase (TRAP)-positive cells in a dose-dependent manner ( Fig. 1a and Supplementary Fig. 1a ). Accordingly, I-BET151 strongly suppressed RANKL-induced expression of osteoclast-related genes such as CTSK (encodes cathepsin K) and ITGB3 (encodes β3 integrin) in human and mouse OCPs ( Fig. 1b and Supplementary Fig. 1b ). Reduced osteoclast formation did not result from changes in cell viability or number, as assessed by MTT assays ( Supplementary Fig. 2a,b ). We next tested whether I-BET151 could inhibit osteoclastogenesis in vivo . I-BET151 strongly inhibited osteoclastogenesis and associated bone erosion in vivo in the TNF-induced supracalvarial osteolysis model ( Fig. 1c ). Consistently, serum TRAP levels were lower in the I-BET151-treated group compared with the vehicle-treated control group ( Fig. 1d ). The reduction in in vivo osteoclastogenesis was further confirmed using histomorphometric analysis to quantify osteoclast numbers and surface area; both osteoclast surface area per bone surface (OcS/BS) and osteoclast numbers per bone surface (NOc/BS) were significantly lower in the I-BET151-treated group ( Fig. 1e ). Collectively, our results show that I-BET151 suppressed osteoclastogenesis in vitro and in vivo . 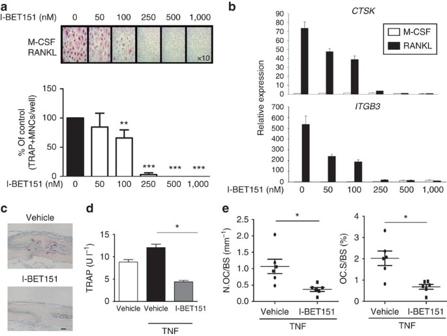Figure 1: I-BET151 inhibits osteoclastogenesis (a) Human OCPs (CD14+monocytes cultured overnight with M-CSF (20 ng ml−1)) were treated with DMSO (vehicle control, labeled 0) or I-BET151 at the indicated concentrations for 1 h before addition of RANKL (40 ng ml−1). After 5 days of culture, TRAP-positive, multinucleated (more than three nuclei) cells were counted in triplicate. The number of osteoclasts generated by RANKL alone is set as 100% for each individual blood donor.Upper panel, representative results from one of more than three experiments.Lower panel,data are shown as mean ±s.e.m. from aggregate data from nine independent donors. **P<0.01, ***P<0.001 by two-way ANOVA. (b) Human OCPs were cultured as inafor 5 days and mRNA was measured using real-time PCR. mRNA levels were normalized relative to GAPDH mRNA. Representative results from at least three independent experiments are shown. (c–e) TNF-induced osteolysis model. TNF (70 μg per kg body weight) was injected over calvarial periosterium for 4 consecutive days, during which time either vehicle control or I-BET151 (40 mg kg−1body weight) in 10 % KLEPTOSE was administrated intraperitoneally (i.p.) once per day. Data shown are from six mice per group. (c) TRAP staining of histological sections obtained from control or I-BET151-treated mice after supracalvarial TNF administration. Scale bar: 100 μm. (d) ELISA measurement of serum TRAP. *P<0.05 by one-way ANOVA. (e) Histomorphometric analysis. Osteoclast number per bone surface (N.Oc BS−1). Osteoclast surface area per bone surface (OcS BS−1). All data are shown as mean ±s.e.m. *P<0.05 byt-test. Figure 1: I-BET151 inhibits osteoclastogenesis ( a ) Human OCPs (CD14 + monocytes cultured overnight with M-CSF (20 ng ml −1 )) were treated with DMSO (vehicle control, labeled 0) or I-BET151 at the indicated concentrations for 1 h before addition of RANKL (40 ng ml −1 ). After 5 days of culture, TRAP-positive, multinucleated (more than three nuclei) cells were counted in triplicate. The number of osteoclasts generated by RANKL alone is set as 100% for each individual blood donor. Upper panel , representative results from one of more than three experiments. Lower panel, data are shown as mean ±s.e.m. from aggregate data from nine independent donors. ** P <0.01, *** P <0.001 by two-way ANOVA. ( b ) Human OCPs were cultured as in a for 5 days and mRNA was measured using real-time PCR. mRNA levels were normalized relative to GAPDH mRNA. Representative results from at least three independent experiments are shown. ( c – e ) TNF-induced osteolysis model. TNF (70 μg per kg body weight) was injected over calvarial periosterium for 4 consecutive days, during which time either vehicle control or I-BET151 (40 mg kg −1 body weight) in 10 % KLEPTOSE was administrated intraperitoneally (i.p.) once per day. Data shown are from six mice per group. ( c ) TRAP staining of histological sections obtained from control or I-BET151-treated mice after supracalvarial TNF administration. Scale bar: 100 μm. ( d ) ELISA measurement of serum TRAP. * P <0.05 by one-way ANOVA. ( e ) Histomorphometric analysis. Osteoclast number per bone surface (N.Oc BS −1 ). Osteoclast surface area per bone surface (OcS BS −1 ). All data are shown as mean ±s.e.m. * P <0.05 by t -test. Full size image I-BET151 protects mice from bone loss in OVX and arthritis To further test the efficacy of inhibiting BET proteins in the treatment of pathological bone loss, we examined the effect of I-BET151 on bone loss in post-ovariectomy (OVX) osteoporosis using a therapeutic experimental design. I-BET151 treatment was started 4 weeks after OVX and continued for 5 weeks ( Fig. 2a ). Microcomputed tomography (μCT) analysis revealed that I-BET151 treatment resulted in significantly increased bone mass relative to vehicle-treated mice ( Fig. 2b,c ). Biomechanical properties of the femurs were assessed by three-point bending, and I-BET151 resulted in significantly increased bone strength compared with vehicle-treated ovariectomized mice ( Fig. 2d ). Histomorphometry showed that I-BET151 decreased osteoclast numbers and surface area, supporting a suppressive effect of I-BET151 on osteoclastogenesis ( Fig. 2e ). Consistent with previous observations [21] , the effects of I-BET in the OVX model with a therapeutic design were similar to those of alendronate ( Supplementary Fig. 3 ), a well-known anti-resorptive reagent that targets osteoclasts with minimal direct effects on osteoblasts [22] . However, we tested the effects of I-BET151 on osteoblast function. At the doses used to suppress osteoclastogenesis in vivo , I-BET151 treatment did not significantly affect mineral apposition rate (MAR) and bone formation rate (BFR) in ovariectomized mice ( Supplementary Fig. 4 ). However, I-BET151 suppressed in vitro osteoblast differentiation at concentrations 5- to 10-fold higher than those required to suppress osteoclastogenesis ( Supplementary Fig. 5 ). Thus, our results suggest that I-BET151 therapeutically increases bone mass in the OVX model by suppressing osteoclastogenesis, but that supra-therapeutic doses have the potential to suppress osteoblast-mediated bone formation. 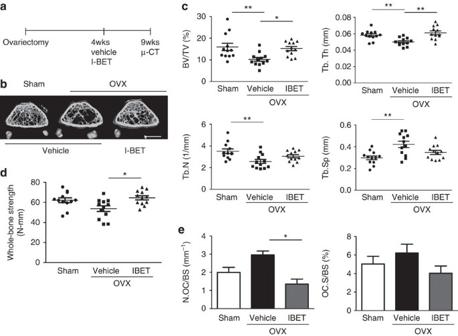Figure 2: I-BET 151 increases bone mass and strength in ovariectomized mice (a) A schematic diagram illustrating the therapeutic experimental design. (b,c) Therapeutic effect of the BET bromodomain protein inhibitor, I-BET151 on post ovariectomy bone loss (n=12 per group). Sham-operated mice (Sham). (b) Representative images showing trabecular architecture by micro-computed tomography (μCT) reconstruction in the distal femurs. Scale bars, 1 mm. (c) μCT measurements for the indicated parameters in distal femurs. Bone volume (BV/TV), trabecular space (Tb.Sp.), trabecular number (Tb.N.) and trabecular thickness (Tb.Th.) were determined by μCT analysis. (d) Three-point bending test of femurs. (e) Histomorphometric analysis of tibia. Osteoclast number per bone surface (N.Oc BS−1). Osteoclast surface area per bone surface (OcS BS−1). All data are shown as mean ±s.e.m. *P<0.05, **P<0.01. One-way ANOVA with apost hocTukey test was performed. Figure 2: I-BET 151 increases bone mass and strength in ovariectomized mice ( a ) A schematic diagram illustrating the therapeutic experimental design. ( b , c ) Therapeutic effect of the BET bromodomain protein inhibitor, I-BET151 on post ovariectomy bone loss ( n =12 per group). Sham-operated mice (Sham). ( b ) Representative images showing trabecular architecture by micro-computed tomography (μCT) reconstruction in the distal femurs. Scale bars, 1 mm. ( c ) μCT measurements for the indicated parameters in distal femurs. Bone volume (BV/TV), trabecular space (Tb.Sp. ), trabecular number (Tb.N.) and trabecular thickness (Tb.Th.) were determined by μCT analysis. ( d ) Three-point bending test of femurs. ( e ) Histomorphometric analysis of tibia. Osteoclast number per bone surface (N.Oc BS −1 ). Osteoclast surface area per bone surface (OcS BS −1 ). All data are shown as mean ±s.e.m. * P <0.05, ** P <0.01. One-way ANOVA with a post hoc Tukey test was performed. Full size image We next tested the effects of I-BET151 in K/BXN serum-induced arthritis, which models the inflammatory effector phase of arthritis and is characterized by joint inflammation and associated bone resorption [23] . I-BET151-treated mice showed decreased joint swelling and inflammation compared with vehicle-treated control mice ( Fig. 3a,b and Supplementary Fig. 6 ). I-BET151-treated mice also showed decreased serum TRAP and decreased osteoclast numbers in periarticular bone ( Fig. 3c–e ). K/BXN serum-induced arthritis is induced by articular immune complexes and is highly dependent on interleukin-1 (IL-1) [24] and chemokine-mediated recruitment of neutrophils [25] . To gain insights into how I-BET151 inhibits arthritic inflammation, we found that I-BET151 suppresses the induction of IL-1 by immune complexes and various inflammatory stimuli, and also attenuates induction of neutrophil chemokines by immune complexes or IL-1 ( Supplementary Fig. 7 ). These results suggest that in the K/BXN arthritis model, I-BET151 potently suppresses bone resorption by a dual action of suppressing inflammation and directly targeting osteoclast differentiation. Taken together, our results establish in vivo efficacy of I-BET151 and suggest that inhibition of BET proteins may represent an effective therapeutic approach for suppressing bone loss. 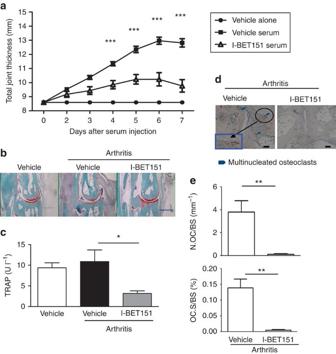Figure 3: I-BET151 attenuates K/BxN serum-induced arthritis. Arthritis was induced in C57BL/6 mice, and I-BET151 was administered as described in Methods. (a) Time course of joint swelling in the presence and absence of I-BET151 treatment. Values are the mean ±s.e.m. of six mice per group. ***P<0.001 by two-way ANOVA. (b) Histology of ankle joints of mice examined 11 days after the first arthritogenic serum injection. Hind paws were fixed and decalcified, and ankle joint sections were prepared and stained with hematoxylin, fast green and Safranin O. Scale bar, 500 μm. (c) Serum TRAP levels were measured 7 days after arthritis induction. *P<0.05 by two-way ANOVA. (d) TRAP staining of histological sections obtained from control or I-BET151 treated arthritic mice. Blue square (inset) shows an enlarged image. Scale bar:100 μm. (e) Histomorphometric analysis. Osteoclast number per bone surface (N.Oc BS−1). Osteoclast surface area per bone surface (OcS BS−1). All data are shown as mean ±s.e.m. **P<0.01 byt-test. Figure 3: I-BET151 attenuates K/BxN serum-induced arthritis. Arthritis was induced in C57BL/6 mice, and I-BET151 was administered as described in Methods. ( a ) Time course of joint swelling in the presence and absence of I-BET151 treatment. Values are the mean ±s.e.m. of six mice per group. *** P <0.001 by two-way ANOVA. ( b ) Histology of ankle joints of mice examined 11 days after the first arthritogenic serum injection. Hind paws were fixed and decalcified, and ankle joint sections were prepared and stained with hematoxylin, fast green and Safranin O. Scale bar, 500 μm. ( c ) Serum TRAP levels were measured 7 days after arthritis induction. * P <0.05 by two-way ANOVA. ( d ) TRAP staining of histological sections obtained from control or I-BET151 treated arthritic mice. Blue square (inset) shows an enlarged image. Scale bar:100 μm. ( e ) Histomorphometric analysis. Osteoclast number per bone surface (N.Oc BS −1 ). Osteoclast surface area per bone surface (OcS BS −1 ). All data are shown as mean ±s.e.m. ** P <0.01 by t -test. Full size image I-BET151 suppresses RANKL-induced NFATc1 expression To test in an unbiased manner for potential targets of I-BET151 that could yield insight into its mechanisms of action, we performed a transcriptomic analysis using high throughput RNA sequencing ( Supplementary Fig. 8 ). I-BET151 suppressed expression of 465 RANKL-induced genes by >50% in two independent donors. These genes are depicted in the heat map in Fig. 4a and listed in Supplementary Table 1 ; Supplementary Figs 9–11 and legends describe our analysis of transcriptomic data. Strikingly, of the 465 I-BET151 targets, 120 genes (26%) are target genes of the master regulator of osteoclastogenesis NFATC1 (ref. 26 ) ( Supplementary Table 2 ), and the expression of NFATC1 itself was suppressed ( Fig. 4a ). NFATc1 drives the early stages of osteoclast differentiation [27] , [28] , [29] , NFATc1-deficient mice develop severe osteopetrosis in vivo [30] , and NFATc1-deficient cells are incapable of differentiating into osteoclasts in vitro [28] , [29] , [31] . Thus, we focused on understanding how I-BET151 suppresses NFATC1 to downregulate osteoclastogenesis. In both human and mouse OCPs, RANKL-induced NFATc1 mRNA and protein expression were inhibited by I-BET151 in a dose-dependent manner ( Fig. 4b,c and Supplementary Fig. 12a,b ). I-BET151 also suppressed RANKL-induced expression of Blimp1, another key regulator of osteoclastogenesis that is induced in part by NFATc1 (refs 32 , 33 ) ( Fig. 4c and Supplementary Fig. 12a ). Downregulation of NFATC1 expression by I-BET151 was not secondary to inhibition of upstream RANK signalling ( Supplementary Fig. 13a ) or induction of known transcriptional repressors of NFATC1 and osteoclast differentiation ( Supplementary Fig. 13b ), suggesting that I-BET151 either directly targets the NFATC1 locus or suppresses an as yet unknown activator of NFATC1 . 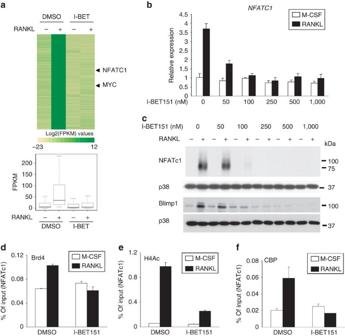Figure 4: I-BET151 inhibitsNFATC1expression. Human OCPs were treated with DMSO or I-BET151 for 1 h, and then cultured with RANKL (40 ng ml−1) for 1 day. (a) Upper panel: heat map of RNA-seq FPKM values for 465 genes which were induced >2-fold by RANKL and whose expression was suppressed by >50% by I-BET151 in two independent donors as shown inSupplementary Fig. 8. Lower panel: box plot depicting FPKM values, (n=2). (b) mRNA was measured using real-time PCR and normalized relative to GAPDH mRNA. Results are shown as means ±s.d. of triplicate determinants. (c) Immunoblot of whole-cell lysates using NFATc1, Blimp1 and p38 antibodies. Same samples were loaded into two gels, and p38 was served as a loading control for each gel. Suppression of NFATc1 expression by I-BET151 was observed in at least 10 independent experiments. Images have been cropped for presentation; full size blots are shown inSupplementary Fig. 18. (d–f) Human OCPs were treated with DMSO (vehicle control) or I-BET151 (500 nM) for 1 h, and RANKL (40 ng ml−1) was added for additional 24 h. Chromatin immunoprecipitation (ChIP) analysis of the NFATC1 promoter for Brd4 (d), acetylated H4 (e) or CBP (f). All data are shown as mean ±s.d. Representative results from at least three independent experiments are shown. Figure 4: I-BET151 inhibits NFATC1 expression. Human OCPs were treated with DMSO or I-BET151 for 1 h, and then cultured with RANKL (40 ng ml −1 ) for 1 day. ( a ) Upper panel: heat map of RNA-seq FPKM values for 465 genes which were induced >2-fold by RANKL and whose expression was suppressed by >50% by I-BET151 in two independent donors as shown in Supplementary Fig. 8 . Lower panel: box plot depicting FPKM values, ( n =2). ( b ) mRNA was measured using real-time PCR and normalized relative to GAPDH mRNA. Results are shown as means ±s.d. of triplicate determinants. ( c ) Immunoblot of whole-cell lysates using NFATc1, Blimp1 and p38 antibodies. Same samples were loaded into two gels, and p38 was served as a loading control for each gel. Suppression of NFATc1 expression by I-BET151 was observed in at least 10 independent experiments. Images have been cropped for presentation; full size blots are shown in Supplementary Fig. 18 . ( d – f ) Human OCPs were treated with DMSO (vehicle control) or I-BET151 (500 nM) for 1 h, and RANKL (40 ng ml −1 ) was added for additional 24 h. Chromatin immunoprecipitation (ChIP) analysis of the NFATC1 promoter for Brd4 ( d ), acetylated H4 ( e ) or CBP ( f ). All data are shown as mean ±s.d. Representative results from at least three independent experiments are shown. Full size image We next investigated mechanisms by which I-BET151 inhibits NFATC1 expression. I-BET151 directly inhibits gene expression by disrupting binding of BET proteins to gene loci [14] . However, using chromatin immunoprecipitation (ChIP) assays, we found that RANKL stimulation resulted in only a modest and not statistically significant recruitment of BET proteins such as Brd4 to the NFATC1 locus ( Fig. 4d ). Although suppression of Brd4 recruitment ( Fig. 4d ) could contribute to the suppression of NFATC1 expression, the weak recruitment of Brd4 suggested that I-BET151 could also regulate NFATC1 expression indirectly, potentially by suppressing the expression of a transcriptional activator required for NFATC1 transcription. Such an indirect mechanism of action was supported by the finding that I-BET151 suppressed RANKL-induced increases in the positive histone mark H4-Ac at the NFATC1 locus ( Fig. 4e ), and, concomitantly, RANKL-induced recruitment to NFATC1 of CBP, a key histone acetyltransferase (HAT) that mediates histone acetylation ( Fig. 4f ). Decreased recruitment of CBP to the NFATC1 promoter suggests that I-BET151 may suppress a RANKL-induced transcription factor that is required to recruit HATs to acetylate histones at NFATC1 . MYC-NFATc1 axis is important for osteoclast differentiation Although the currently appreciated important transcriptional regulators of osteoclastogenesis [34] are not known BET targets ( Fig. 4a and Supplementary Fig. 13 ), the transcription factor MYC is dependent on BET proteins [18] , [35] and was suggested to play a role in osteoclastogenesis in RAW267.4 cells and mouse osteoclasts [36] , [37] ; however, mechanisms by which MYC regulates osteoclastogenesis remain to be elucidated. Strikingly, analysis of our transcriptomic data showed that 73 out of 465 (16%) of I-BET targets correspond to MYC target genes ( Supplementary Fig. 10 ), that MYC-dependent cellular processes were suppressed by I-BET151 ( Supplementary Figs 9 and 11 ) and that MYC- and NFAT-target genes overlap ( Supplementary Fig. 10 ). These results support the idea that a MYC-NFATC1 axis is important for osteoclastogenesis and thus we addressed the role of MYC in our system. RANKL-induced MYC ( Fig. 5a ) with similar kinetics as induction of NFATc1 ( Supplementary Fig. 14 ). I-BET151 abrogated RANKL-induced MYC expression in human and mouse OCPs ( Figs 4a and 5a and Supplementary Fig. 15 ). To examine the role of MYC in human OCPs, we treated cells with an MYC inhibitor 10058-F4 (ref. 38 ) or knocked down MYC expression using siRNAs. Inhibition of MYC suppressed osteoclast differentiation ( Fig. 5b ). We then tested whether MYC regulates the expression of NFATC1 . An MYC inhibitor 10058-F4 inhibited RANKL-induced NFATC1 mRNA and protein expression in a dose-dependent manner in human and mouse OCPs ( Fig. 5c,d and Supplementary Fig. 16 ). Consistently, siRNA-mediated knockdown of MYC inhibited osteoclastogenesis and RANKL-induced NFATc1 expression ( Supplementary Fig. 17 ). Furthermore, ChIP assays showed that RANKL stimulation induced recruitment of MYC to the NFATC1 promoter, supporting direct regulation of NFATC1 by MYC ( Fig. 5e ). This RANKL-induced occupancy of MYC at the NFATC1 promoter was effectively suppressed by I-BET151 ( Fig. 5e ). Inhibition of MYC decreased RANKL-induced H4-Ac at the NFATC1 promoter ( Fig. 5f ) in a manner parallel to decreased H4-Ac after I-BET151 treatment ( Fig. 4e ). These results indicate that MYC is required for the induction of H4-Ac at the NFATC1 promoter. Accordingly, MYC inhibition resulted in similar decreases in RANKL-induced recruitment of CBP to NFATC1 ( Fig. 5g ). These results establish inhibition of MYC as a mechanism by which I-BET151 regulates NFATC1 and support a role for MYC in osteoclastogenesis. We previously reported that the expression of NFATC1 protein is increased in synovial OCPs of rheumatoid arthritis (RA) patients [39] , which have a higher potential for differentiating into osteoclasts [40] . To investigate a potential role for MYC in vivo , we first examined MYC expression in RA synovial OCPs. Quantitative RT-PCR analysis showed significantly increased MYC expression in RA synovial CD14 + OCPs relative to disease controls and a parallel increase in NFATC1 mRNA ( Fig. 5h ). These results suggested a role for MYC in osteoclastogenesis in inflammatory settings, which we further investigated using the TNF-induced supracalvarial osteolysis model. Similar to I-BET151 treatment, the MYC inhibitor 10058-F4 suppressed TNF-induced serum TRAP ( Fig. 5i ) and significantly reduced both osteoclast surface area per bone surface (OcS/BS) and osteoclast numbers per bone surface (NOc/BS) ( Fig. 5j ). Taken together, these results reveal MYC as an important factor in osteoclastogenesis and suggest targeting MYC as a new therapeutic strategy to control bone resorption. 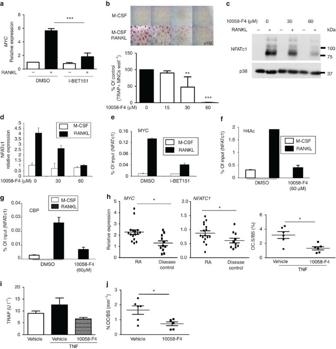Figure 5: I-BET151 suppresses RANKL-induced MYC expression. (a) Human OCPs were treated with DMSO or I-BET151 at the indicated concentrations for 1 h, and then cultured with RANKL (40 ng ml−1) for 1 day (n=4). Analysis of expression of MYC mRNA by real-time PCR. All data are shown as mean±s.e.m. ***P<0.001 by One-way ANOVA. (b) (n=4), osteoclastogenesis assay. Human OCPs were cultured with either DMSO (vehicle control) or 10058-F4 at the indicated doses for 1 h before RANKL stimulation, and TRAP-positive multinucleated (more than three nuclei) cells were counted 5 days after RANKL addition.Upper panel, representative results obtained from one donor are shown.Lower panel,data are shown as means±s.e.m. (c,d) Cells were cultured with 10058-F4 at the indicated doses for 1 h, and RANKL was then added for 2 days. (c) Immunoblot of whole-cell lysates with NFATc1 and p38 antibodies. Images have been cropped for presentation; full-size blots are shown inSupplementary Fig. 18. (d)NFATc1mRNA was measured by real-time PCR. mRNA levels were normalized to the expression of GAPDH. (e–g) ChIP analysis for MYC (e), acetylated H4 (f), or CBP (g) at theNFATC1promoter in human OCPs. Representative results from three independent experiments are shown. All data are shown as mean ±s.d. (h) MYC and NFATC1 expression in RA synovial macrophages. mRNA from synovial CD14+cells from rheumatoid arthritis patients (n=16) or sero-negative arthritis disease control patients (n=11) was measured using real-time PCR. mRNA levels were normalized relative to the expression of GAPDH. All data are shown as mean ±s.e.m. *P<0.05; byt-test. (i,j) TNF-induced supracalvareal osteolysis;n=6. TNF (83 μg per kg body weight) was injected over calvarial periosterium for five consecutive days, and either vehicle (DMSO) or 10058-F4 (30 mg kg−1) was administrated intraperitoneally (i.p.) once per day. (i) The concentration of serum TRAP measured by ELISA. (j) Histomorphometric analysis of calvaria from either vehicle or 10058-F4-treated mice; osteoclast number per bone surface (N.Oc BS−1) and osteoclast surface area per bone surface (OcS BS−1). All data are shown as mean±s.e.m. *P<0.05 byt-test. Figure 5: I-BET151 suppresses RANKL-induced MYC expression. ( a ) Human OCPs were treated with DMSO or I-BET151 at the indicated concentrations for 1 h, and then cultured with RANKL (40 ng ml −1 ) for 1 day ( n =4). Analysis of expression of MYC mRNA by real-time PCR. All data are shown as mean±s.e.m. *** P <0.001 by One-way ANOVA. ( b ) ( n =4), osteoclastogenesis assay. Human OCPs were cultured with either DMSO (vehicle control) or 10058-F4 at the indicated doses for 1 h before RANKL stimulation, and TRAP-positive multinucleated (more than three nuclei) cells were counted 5 days after RANKL addition. Upper panel , representative results obtained from one donor are shown. Lower panel, data are shown as means±s.e.m. ( c , d ) Cells were cultured with 10058-F4 at the indicated doses for 1 h, and RANKL was then added for 2 days. ( c ) Immunoblot of whole-cell lysates with NFATc1 and p38 antibodies. Images have been cropped for presentation; full-size blots are shown in Supplementary Fig. 18 . ( d ) NFATc1 mRNA was measured by real-time PCR. mRNA levels were normalized to the expression of GAPDH. ( e – g ) ChIP analysis for MYC ( e ), acetylated H4 ( f ), or CBP ( g ) at the NFATC1 promoter in human OCPs. Representative results from three independent experiments are shown. All data are shown as mean ±s.d. ( h ) MYC and NFATC1 expression in RA synovial macrophages. mRNA from synovial CD14 + cells from rheumatoid arthritis patients ( n =16) or sero-negative arthritis disease control patients ( n =11) was measured using real-time PCR. mRNA levels were normalized relative to the expression of GAPDH. All data are shown as mean ±s.e.m. * P <0.05; by t -test. ( i , j ) TNF-induced supracalvareal osteolysis; n =6. TNF (83 μg per kg body weight) was injected over calvarial periosterium for five consecutive days, and either vehicle (DMSO) or 10058-F4 (30 mg kg −1 ) was administrated intraperitoneally (i.p.) once per day. ( i ) The concentration of serum TRAP measured by ELISA. ( j ) Histomorphometric analysis of calvaria from either vehicle or 10058-F4-treated mice; osteoclast number per bone surface (N.Oc BS −1 ) and osteoclast surface area per bone surface (OcS BS −1 ). All data are shown as mean±s.e.m. * P <0.05 by t -test. Full size image Cytokines, receptors, signalling pathways and transcription factors that regulate osteoclastogenesis have been extensively characterized [1] , [41] , resulting in the identification of therapeutic targets, such as RANKL and NFATC1, for the treatment of pathological bone resorption [2] , [3] , [4] . Emerging evidence suggests that chromatin states and related epigenetic mechanisms that control how information encoded in DNA is expressed play an important role in osteoclastogenesis [6] , [7] , [31] . As many chromatin regulators are enzymes or ‘readers’ that can be targeted by conventional small-molecule approaches [11] , this opens up new therapeutic opportunities for suppression of osteoclastogenesis and pathologic bone resorption. In this study, we show that I-BET151 inhibits osteoclast differentiation and suppresses in vivo osteoclastogenesis and pathologic bone resorption in three distinct disease models: TNF-induced inflammatory osteolysis, inflammatory arthritis and post ovariectomy low oestrogen-mediated osteoporosis. Mechanistically, I-BET151 inhibited expression of the master osteoclast regulator NFATC1 by suppressing expression and recruitment of its upstream regulator MYC. MYC was elevated in rheumatoid arthritis synovial macrophages and its induction by RANKL was important for osteoclastogenesis and TNF-induced bone resorption. These results highlight the importance of an I-BET151-inhibited MYC-NFATC1 axis in osteoclastogenesis and pathologic bone resorption. Epigenetic mechanisms contribute to regulation of the expression of genes, and therapies targeting epigenetic marks including DNA methylation and histone modifications such as acetylation and methylation show therapeutic efficacy in several diseases and various disease models [11] , [12] . In preclinical studies, the related compounds I-BET151 and I-BET762, and JQ1, appear safe and highly efficacious in treatment of NUT midline carcinoma, acute myeloid leukemia and multiple myeloma, [15] , [18] , [42] and I-BET762 (ref. 14 ) is currently in clinical trials (clinicaltrials.gov reference NCT01587703). We have demonstrated therapeutic efficacy of I-BET151, a compound that targets an epigenetic mechanism important for osteoclastogenesis, in increasing bone mass and strength in the standard post OVX model of osteoporosis. While our manuscript was under revision, the related BET inhibitor JQ1 was reported to suppress osteosarcoma-mediated bone remodelling by suppressing the function of both osteoclasts and osteoblasts [43] . As we have found that 5- to 10-fold higher concentrations of I-BET151 are required to suppress osteoblast differentiation than osteoclastogenesis ( Supplementary Figs 1 and 5 ), the differences in results, namely the lack of suppression of osteoblast function in vivo in our study, may be explained by differences in dosing or pharmacokinetics of these two BET inhibitors. Alternatively, it is possible that distinct pathogenic mechanisms in inflammatory or low oestrogen-mediated bone loss versus tumour-mediated bone remodelling [5] result in differential responses to BET inhibitors. Overall our results in the post-ovariectomy model that I-BET151 suppressed osteoclastogenesis and bone resorption but minimally affected bone formation suggest a therapeutic window in which I-BET151 can exert beneficial effects on bone mass. I-BET151 effectively suppressed osteoclastogenesis and pathologic bone resorption in inflammatory disease models. Inflammatory bone resorption can be refractory to established antiresorptive therapies [3] , [44] , such as bisphosphonates, that target osteoclasts. In the K/BxN arthritis model, I-BET151 suppressed inflammation as well as bone resorption. Thus, I-BET151 offers the advantage of both suppressing inflammation, thus indirectly dampening osteoclastogenesis and directly suppressing osteoclast differentiation. BET inhibitors have been shown to suppress induction of inflammatory secondary response genes by bacterial lipopolysaccharide (LPS) [14] and we have extended this work to show that I-BET151 suppresses immune complex- and IL-1-induced expression of cytokines and neutrophil chemoattractants that are important for inflammatory arthritis. The combined effect of suppressing inflammation and osteoclastogenesis suggests targeting BET proteins may be effective in suppressing pathological bone resorption that occurs in inflammatory settings. BET inhibitors may have different therapeutic targets in various diseases [11] . One such target is MYC and BET inhibitors have therapeutic applications in MYC-driven disorders, which have otherwise been refractory to various therapeutic strategies to target MYC. Our results suggest that in osteoclasts I-BET151 works at least in part by suppressing MYC and targeting a newly described MYC-NFAT axis important for osteoclastogenesis. MYC has been previously implicated in osteoclastogenesis but the mechanism by which MYC regulates osteoclastogenesis was not clear [36] , [37] . Our investigation of mechanisms of I-BET151 action revealed a role for MYC in osteoclast differentiation and inflammatory bone resorption. One mechanism of MYC action was direct binding to and activation of NFATC1 expression, although it is possible that MYC also promotes osteoclastogenesis by additional mechanisms that remain to be investigated. In summary, our results on the importance of BET proteins and MYC in osteoclastogenesis open new lines of investigation in the understanding and therapeutic targeting of pathological bone resorption. Mice and analysis of bone phenotype Six-week-old female C57BL/6 were purchased from The Jackson Laboratory (Bar Harbor, ME). All animal experiments were approved by the Hospital for Special Surgery Institutional Animal Care and Use Committee (IACUC). All animals were randomly assigned into experimental groups. For ovariectomy (OVX)-induced bone loss model, 16-week-old sham-operated or ovariectomized CD-1 mice were purchased from Charles River Laboratory (Wilmington, MA). I-BET151 was prepared in 10% KLEPTOSE (Roquette Pharma) following the manufacturer’s instructions. Ovariectomized mice were randomly divided into two groups (vehicle versus I-BET; n =12 per group). To analyse the therapeutic effect of I-BET151, either vehicle or I-BET151 (30 mg kg −1 ) was administrated intraperitoneally (i.p.) once per day beginning 4 weeks after surgery. I-BET151 or vehicle injection was continued for 5 weeks. After 5-week treatment, femurs were isolated and μ-CT analysis [45] was performed at the Musculoskeletal Repair and Regeneration Core Center in Hospital for Special Surgery as described previously [46] , and all samples were included in the analysis conducted in a blinded manner. For arthritis experiments, K/BxN serum pools were prepared as described previously [47] . Arthritis was induced by intraperitoneal injection of 100 μl of K/BxN serum on days 0 and 2. Arthritic mice were divided into two groups (vehicle versus I-BET151; n =9 mice per group) and were administered vehicle or I-BET151 (40 mg kg −1 ) once on days 0 and 2 and twice per day from day 3 to day 6. Control group ( n =9) only received vehicle but not arthritic serum. The severity of arthritis was monitored by measuring the thickness of both the wrist and ankle joints using dial-type calipers (Bel-Art Products). For each animal, joint thickness was calculated as the sum of the measurements of both wrists and both ankles. Joint thickness was represented as the average for every treatment group. For inflammatory osteolysis experiments, we used an established mouse model, the TNF-induced supracalvarial osteolysis model [48] with minor modifications. In brief, TNF was administrated daily at the doses indicated in the figure legends to the calvarial periosteum of mice for four to five consecutive days. The mice were then killed for the collection of serum and calvarial bones for sectioning. For histopathologic assessment, mice were killed, and the hind paws and calvarial bones were harvested and fixed in 4% paraformaldehyde for 2 days. These samples were decalcified with 10% neutral buffered EDTA (Sigma-Aldrich) and embedded in paraffin. To assess osteoclastogenesis and bone resorption, sections were stained with TRAP (tartrate-resistant acid phosphatase) and hematoxylin for osteoclast visualization, and histomorphometric analysis was performed with the BioQuant image analysis system (Nashville, TN, USA) using standard procedures [49] . Osteoclasts were identified as TRAP + cells that were multinucleated and adjacent to bone. As markers for osteoclast formation and bone resorption, serum TRAP5b was measured with the RatLaps enzyme immunoassay (EIA) kit (Immunodiagnostic Systems) following the manufacturer’s instructions. Methods of bone mineralization and osteoblast differentiation analysis are shown in Supplementary Information . Three-point bending test The whole bone strength of the femur was measured in bending. Femurs were loaded in three-point bending to failure [50] . The bones were positioned with the posterior aspect resting on the supports (6 mm span), and the load was applied to the anterior mid-diaphysis at a rate of 0.1 mm s −1 (Bose Enduratec). The bending strength (maximum moment) and stiffness were determined from the applied load and displacement data. All samples were included in the analysis conducted in a blinded manner. Reagents Human and murine M-CSF, sRANKL and TNF were purchased from Peprotech (Rocky Hill, NJ). I-BET was synthesized by GlaxoSmithKline (UK) as previously described [15] , [51] , [52] . An MYC inhibitor 10058-F4 was purchased from Sigma-Aldrich. The MTT assay kit was purchased from Roche, and cell viability was measured following the manufacturer’s instructions. The antibodies (1:1,000) used for immunoblotting are as follows: NFATc1(BD Pharmagen; 556602); c-myc and p38 (Santa Cruz Biotechnology; sc-764 and sc535); Lamin B (Abcam; ab16048); phospho-ERK, IκBα, phospho-p38 and Blimp1 (Cell Signaling; 9101, 9242, 9215, 9115). Cell culture Peripheral blood mononuclear cells were obtained from blood leukocyte preparations purchased from the New York Blood Center by density gradient centrifugation with Ficoll (Invitrogen, Carlsbad, CA) using a protocol approved by the Hospital for Special Surgery Institutional Review Board. Monocytes were obtained from peripheral blood using anti-CD14 magnetic beads, as recommended by the manufacturer (Miltenyi Biotec Auburn, CA). Monocyte-derived osteoclast precursors (OCPs) that express RANK were obtained by culturing for 1 day with 20 ng ml −1 of M-CSF (Peprotech) in α-MEM medium (Invitrogen) supplemented with 10 % fetal bovine serum (FBS, Hyclone), and the purity of monocytes was >97%, as verified by flow cytometric analysis. Osteoclast differentiation Human CD14 + cells were incubated with 20 ng ml −1 of M-CSF for 1 day to generate OCPs. For human osteoclastogenesis assays, cells were added to 96-well plates in triplicate at a seeding density of 5 × 10 4 cells per well. Osteoclast precursors were incubated with 20 ng ml −1 of M-CSF and 40 ng ml −1 of human soluble RANKL for five additional days in α-MEM supplemented with 10 % FBS. Cytokines were replenished every 3 days. On day 6, cells were fixed and stained for TRAP using the Acid Phosphatase Leukocyte diagnostic kit (Sigma) as recommended by the manufacturer. Multinucleated (>3 nuclei), TRAP-positive osteoclasts were counted in triplicate wells. For mouse osteoclastogenesis, bone marrow (BM) cells were flushed from femurs of mice and cultured with murine M-CSF (20 ng ml −1 , Peprotech) on petri dishes in α-MEM supplemented with 10% FBS after lysis of RBCs using ACK lysis buffer (Cambrex, Walkersville, MD). Then, the non-adherent cell population was recovered the next day and cultured with murine M-CSF (20 ng ml −1 ) for three additional days. We defined this cell population as mouse OCPs. For murine osteoclastogenesis assays, we plated 2 × 10 4 OCPs per well in triplicate wells on a 96-well plate and added M-CSF and RANKL (100 ng ml −1 ) for an additional 6 days, with exchange of fresh media every 3 days. Imaging was performed with a × 10 objective. Gene expression analysis For real-time PCR, DNA-free RNA was obtained using the RNeasy Mini Kit from QIAGEN with DNase treatment, and 0.5 μg of total RNA was reverse transcribed using a First Strand cDNA Synthesis kit (Fermentas, Hanover, MD). Real-time PCR was performed in triplicate using the iCycler iQ thermal cycler and detection system (Applied Biosystems, Carlsbad, CA) following the manufacturer’s protocols. Expression of the tested gene was normalized relative to the levels of GAPDH. RNA sequencing Total RNA was first extracted using RNeasy mini kit (Qiagen). True-seq sample preparation kits (Illumina) were then used to purify poly-A transcripts and generate libraries with multiplexed barcode adaptors. All samples passed quality control analysis on a Bioanalyzer 2100 (Agilent). Paired-end reads (50 × 2 cycles, ~75 × 10 6 reads per sample) were obtained on an Illumina HiSeq 2500/1500 in the Weill Cornell Medical College Genomics Resources Core Facility. The TopHat program (v 1.2.0) was used to align the reads to the UCSC Hg19 human reference genome, while the Cufflinks program (v. 0. 93) allowed for measurements of transcript abundance (represented by Fragments Per Kilobase of exon model per Million mapped reads (FPKM)). Genes and transcripts with FPKM values <5 were not included in the analysis. Pearson correlation analysis and heatmaps were generated using R (3.0.2). The RNA sequencing data have been deposited to the Sequence Read Archive ( http://www.ncbi.nlm.nih.gov/sra/ ) and assigned study number SRP047069. Chromatin immunoprecipitation ChIP was performed as previously described [14] . In brief, 2 × 10 7 human primary OCPs were fixed by adding formaldehyde directly to the medium to a final concentration of 1 % for 5 min. Cells were harvested, washed and lysed. Chromatin was sheared by sonication to a length of ~500 base pairs using a Bioruptor sonicator (Diagenode). Sheared chromatin was precleared and then immunoprecipitated with antibodies; c-myc (Abcam; ab56), Brd4 (Bethyl Lab; A301-985A), pan acetyl-H4 (Millipore; 06-866), and CBP (Abcam; ab2832). Immune complexes were subsequently collected and washed, and DNA crosslinking was reversed by heating at 65 °C overnight. Following proteinase K digestion, DNA was recovered using the PCR purification kit (Qiagen) and real-time PCR was performed to detect the occupancy of target proteins. Signals obtained from the ChIP are divided by signals obtained from an input sample. This input sample represents the amount of chromatin used in the ChIP. The primer sequences are listed in Supplementary Table 3 . Statistical analysis All statistical analyses were performed with Graphpad Prism 5.0 software using the two-tailed, unpaired t -test (two conditions), one-way or two-way ANOVA for multiple comparisons (more than two conditions) with post hoc Tukey test. P <0.05 was taken as statistically significant. How to cite this article: Park-Min, K.-H. et al. Inhibition of osteoclastogenesis and inflammatory bone resorption by targeting BET proteins and epigenetic regulation. Nat. Commun. 5:5418 doi: 10.1038/ncomms6418 (2014).